Orbital resolution of molecules covalently attached to a clean semiconductor surface Understanding the chemical and electronic nature of molecules attached to semiconductors is of great importance in the study of molecule-based electronic devices. Resolving individual molecular orbitals using scanning tunnelling microscopy is a straightforward approach but remains challenging on the semiconductor surfaces because of their highly reactive dangling bonds. Here we show that hybridized molecular orbitals of pyridazine molecules covalently attached to Ge(100) surfaces can be resolved by scanning tunnelling microscopy. Pyridazine binds to Ge(100) through single/double dative bond(s) and presents two types of features with three and four lobes. These features resemble the lowest unoccupied molecular orbitals of free pyridazine, which are hybridized by the surface states in the adsorbed state. The adsorbing sites, binding mechanisms, orientations and electronic properties of the adsorbed molecules are convincingly determined. Our results indicate that orbital resolution of molecules covalently attached to semiconductors is accessible despite of their high reactivity. The fabrication of organic molecules on semiconductor surfaces has recently stimulated increasing interest for potential applications in molecule-based electronics devices [1] , [2] , [3] . The interest arises from the possible incorporation of organic molecules of tuneable chemical and electronic properties into existing semiconductor-based microelectronic technologies [4] . Such incorporations require a detailed understanding of the chemical and electronic nature of the designed organic/semiconductor junctions [5] . Unfortunately, semiconductor surfaces usually have highly reactive and unevenly distributed dangling bonds that likely react with an organic molecule in multiple reaction pathways, which complicate the characterizations using various surface tools [6] , [7] . While spectroscopic surface tools reveal information only on an ensemble of adsorbed molecules, scanning tunnelling microscopy (STM) is a powerful tool for this task because of its capability of capturing geometric and electronic information, particularly the orbital details, of individual adsorbates on a molecular/atomic scale. Although an orbital is not a quantum observable, but its energy level and electron density contribute to the tunnelling conductance, thus can be spatially resolved by STM [8] . It has been demonstrated on other surfaces that once molecular orbitals are resolved by STM, many chemical reaction mechanisms and inherent electronic properties of single molecules can be directly and reliably elucidated [9] , [10] , [11] , [12] , [13] . However, orbital resolution is rather difficult to achieve because of the need of delicate STM tip modification [14] , [15] , [16] , [17] , [18] , [19] , [20] and substrate preparation [12] , [15] , [21] , [22] . In addition, most molecules undergo addition or dissociation on semiconductor surfaces, resulting in blurred profiles during STM scanning, thus losing insightful electronic details such as orbitals [23] . Therefore, spatially resolving the orbitals of molecules on clean semiconductors is still challenging but highly desirable. Here we demonstrate that orbital resolution can be achieved for a planar molecule pyridazine attached to a clean semiconductor surface through covalent bonds. Two types of molecular features with nodal planes are observed and assigned to pyridazine binding to Ge(100) through single/double N–Ge dative bond(s). The captured orbitals resemble the lowest unoccupied molecular orbital (LUMO) of free pyridazine, which is hybridized by surface states and becomes occupied, thus visible in the adsorbed state. The binding mechanisms, orientations and electronic properties of the adsorbed molecules are convincingly determined based on the orbital-resolvable STM images. STM images of adsorbed molecules We investigated pyridazine (C 4 H 4 N 2 ), a six-membered heterocycle with two N atoms, on Ge(100) surfaces, which are composed of Ge–Ge dimers. Ge(100) is chosen as the substrate because of its higher electron mobility than Si and the candidature for the next generation of semiconductor materials. 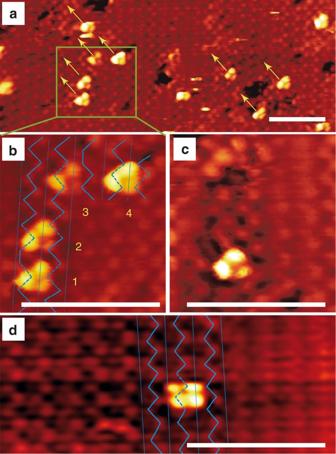Figure 1: Constant current scanning tunnelling microscopy images of pyridazine adsorbed on a clean Ge(100) surface. (a) Filled-state images of pyridazine adsorbed on a clean Ge(100) surface. The yellow arrows mark the uniform orientation of clover features with three leaves. Bias: −2.0 V. (b) Zoomed-in clover features in the green rectangle ina. The zigzag chains inbanddsketch the up Ge dimer atoms of Ge(100). (c) A clover feature at a bias of −0.5 V. (d) A lucky-clover feature with four leaves on a dimer row. Bias: −2.0 V. Tunnelling current for all images: 300 pA. Scale bar, 4 nm. [24] Figure 1 presents filled-state STM images of pyridazine adsorbed on a clean Ge(100) surface at room temperature. Dosing pyridazine onto Ge(100) produces two types of protrusions. Figure 1a shows the major type of adsorption features. Unlike the protrusions without nodal planes that are usually in conventional STM images, here, each molecule of this type appears as a ‘clover’—with three leaves separated by nodal planes. Two leaves are almost equal in size and larger than the third one, rendering the ‘clover’ asymmetric. In addition, these clover features are of a uniform azimuth angle (marked by arrows). Because the substrate atoms exhibit a normal spherical appearance, the possible STM tip illusion can be excluded, and these clover features provide additional structural information. By sketching up-dimer atoms of clean Ge(100) before adsorption, the centre of each ‘clover’ is located in dimer troughs as illustrated in Fig. 1b . In addition, the locations of these ‘clovers’ can be further divided into two groups: the centres of molecules 1 and 2 are at the left side of the trough line, whereas 3 and 4 located on the trough line. The similar clover appearance at −0.5 V in Fig. 1c indicates that the clover appearance is bias insensitive under STM in the range of −2 to 0 V. Figure 1: Constant current scanning tunnelling microscopy images of pyridazine adsorbed on a clean Ge(100) surface. ( a ) Filled-state images of pyridazine adsorbed on a clean Ge(100) surface. The yellow arrows mark the uniform orientation of clover features with three leaves. Bias: −2.0 V. ( b ) Zoomed-in clover features in the green rectangle in a . The zigzag chains in b and d sketch the up Ge dimer atoms of Ge(100). ( c ) A clover feature at a bias of −0.5 V. ( d ) A lucky-clover feature with four leaves on a dimer row. Bias: −2.0 V. Tunnelling current for all images: 300 pA. Scale bar, 4 nm. Full size image The minor adsorption state is shown in Fig. 1d . This state is rare and less stable than the clover feature, and we only observed a few incomplete profiles. The state consists of four leaves separated by cross-like nodal planes, clearly distinguishing it from the three-leaved ‘clovers’, and we call them ‘lucky-clovers’. The centre of the lucky-clover feature is on top of a dimer, which is different from the three-leaved ‘clovers’. Experimentally, we observed two types of adsorbing features of pyridazine with nodal planes on Ge(100) during in situ dosing. Such a good resolution heavily depends on the tip condition, as we obtained conventional resolution if we scanned the sample after dosing. STM tips were reported to offer better resolution when the tip apexes are modified by CO or organic molecules [14] , [17] , [18] , [20] . In our experiments, the onset of better resolution is related to a molecule dropping and reattaching process by tracing the tip state ( Supplementary Fig. 1 ). The modification of STM tips by molecules is facilitated during in situ dosing because biased tips tend to attract molecules during scanning. More experiments to survey the effect of in situ dosing are in progress. Adsorption geometries We performed density functional theory DFT calculations to interpret the adsorption structures and gain insight into the binding mechanisms. Pyridazine contains two adjacent N atoms, and has many thermodynamically allowed pathways when reacting with Ge(100), such as N–Ge single and double dative bonding, [4+2] and [2+2] cycloadditions ( Supplementary Fig. 2 ). Conventional STM images without nodal planes may provide some information on binding sites, but not detailed bonding configurations. For example, the clover feature might be assigned to any adsorption structure of pyridazine in dimer troughs, whereas the lucky-clover feature could be related to any products on dimer rows. In contrast, by correlating our STM images in high resolution with theoretical simulations at different biases ( Supplementary Fig. 3 ), it is possible to convincingly identify the adsorption structures among many candidates (in Supplementary Fig. 2 ). We observed that only the NN-dative model in Fig. 2a produces the lucky-clover feature ( Fig. 2c,d ), with an excellent consistency in shape, number of leaves, orientation and locations. In this model, pyridazine binds to a Ge–Ge dimer through two N–Ge dative bonds. Similarly, only the simulated STM image of N-dative ( Fig. 2b ) well matches the clover feature at −2.0 V ( Fig. 2e,f ) and −0.5 V ( Fig. 2g,h ). In the N-dative state, pyridazine binds to a dimer atom through a single N–Ge dative bond, on either the left or the right side of a trough. In Fig. 2b , pyridazine binds to the right dimer of a trough, corresponding to molecules 1 and 2 ( Fig. 1b ). Pyridazine could also bind to the left dimer of the trough, appearing as molecules 3 and 4 with their centres on the left side of the trough lines in STM images. The uniform orientation of all the ‘clovers’ suggests that their ring planes are tuned and directionally aligned by a lateral electric field. This field is likely to be induced by the non-axisymmetric potential distribution of the sharp STM tip after molecular modification because both lateral and vertical electric fields produced by STM tips are able to significantly change the tilt angle, orientation and location of adsorbed polar molecules [25] , [26] , [27] . The sizes of all the adsorbed features in the STM images are larger than our theoretical prediction, which might be ascribed to the limitation of the simulation method [8] because it does not consider the tip effect. In addition, our high resolution electron energy loss spectroscopy (HREELS) spectra also confirm that pyridazine binds to Ge(100) dimers only through N–Ge bond(s), and the aromaticity of pyridazine is retained on adsorption ( Supplementary Fig. 4 and Supplementary Table 1 ). Thermodynamically, the adsorption energies of NN-dative (105 kJ mol −1 ) and N-dative (120 kJ mol −1 ) are the two greatest among all the candidates, in accordance with preference of N-dative bonding for N-containing heterocycles reacting with Ge(100) [28] , [29] . Kinetically, the dative binding is favourable without barriers. Thus, we conclude that NN-dative and N-dative are two adsorption products observed under STM. The discrepancy in adsorption energies also explains why the most stable N-dative state dominates over the less stable lucky-clover feature. 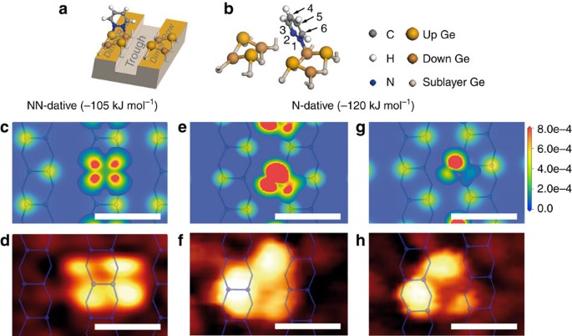Figure 2: Theoretically predicted adsorption structures and simulated STM images. (a,b) Geometric structures of pyridazine binding to Ge dimer atoms through double N–Ge bonds (a) or a single N–Ge bond (b). (c) Simulated STM images ofaat a bias of −2.0 V. (d) STM image of the lucky-clover feature adapted fromFig. 1d. (e) Simulated STM images ofbat biases of −2.0 V and (g) −0.5 V. (f) STM image of the clover feature adapted fromFig. 1bat biases of −2.0 V and (h) −0.5 V (fromFig. 1c). All scale bar, 0.8 nm. The colour bar legends are in the unit of e Å−3. Figure 2: Theoretically predicted adsorption structures and simulated STM images. ( a , b ) Geometric structures of pyridazine binding to Ge dimer atoms through double N–Ge bonds ( a ) or a single N–Ge bond ( b ). ( c ) Simulated STM images of a at a bias of −2.0 V. ( d ) STM image of the lucky-clover feature adapted from Fig. 1d . ( e ) Simulated STM images of b at biases of −2.0 V and ( g ) −0.5 V. ( f ) STM image of the clover feature adapted from Fig. 1b at biases of −2.0 V and ( h ) −0.5 V (from Fig. 1c ). All scale bar, 0.8 nm. The colour bar legends are in the unit of e Å −3 . Full size image Orbital resolution In a simplified STM tunnelling mode without consideration of the tip and tunnelling channels, constant current images map the local density of states (DOS) or accumulation of orbitals of the pyridazine/Ge(100) system [8] . 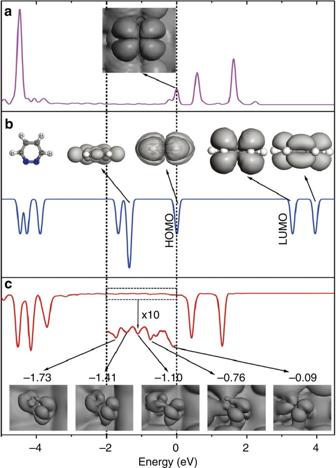Figure 3: Density of states (DOS) curve and orbitals of N-dative and NN-dative configurations. (a) Partial DOS curve of pyridazine and the highest occupied molecular orbital (HOMO, inset) of the NN-dative structure. (b) DOS of free pyridazine. The insets show pyridazine’s geometric structure and frontier orbitals. (c) Partial DOS curve of pyridazine of the N-dative structure, and the major frontier orbitals of the N-dative structure between −2 and 0 eV. The isovalue to plot the electron density isosurfaces of all orbitals is 1 × 10−4e Å−3. The two vertical dash lines indicate the scanning tunnelling microscopy-resonating bias range from −2 to 0 eV. The energies refer to the valence band maximum of each model as zero. Figure 3a shows the calculated partial DOS curve of pyridazine in the NN-dative model. One distinct peak (orbital) is present in the STM resonance range (−2 to 0 eV, relative to the valence band maximum of each adsorption model hereafter). It is this orbital that exhibits the lucky-clover feature. Experimentally, a d I /d V measurement above the molecule could be useful to further confirm the existence of this exclusive peak in the real resonance range. Unfortunately, this information was not obtained due to the limitation of our instrumental functionality. Although this orbital conceptually belongs to the molecule/Ge(100) system due to existence of covalent bonding between the molecule and substrate, its source could be traced by comparing it with the molecular orbitals of free pyridazine. Compared with the frontier orbitals of the free molecule in Fig. 3b , this ‘lucky-clover’ orbital (in the inset of Fig. 3a ) mainly originates from the LUMO of pyridazine. DOS curves and charge analysis suggest complex charge transfer behaviours in NN-dative, including the N atom donating its lone pair electrons to the binding Ge atom and this Ge atom back-donating electrons to the LUMO of pyridazine. The LUMO of free pyridazine becomes occupied in the adsorbed state and is visible in the filled-state STM images. However, two N–Ge dative bonds in NN-dative eliminate dangling bonds of the binding dimer, thus alleviating the coupling of the LUMO of pyridazine with the surface states. The total DOS curve of the NN-dative model (not shown here) indicates that although there are abundant surface states (from other unreacted dimers) between −2 and 0 eV, they are spatially isolated and do not couple with the LUMO of pyridazine. Figure 3: Density of states (DOS) curve and orbitals of N-dative and NN-dative configurations. ( a ) Partial DOS curve of pyridazine and the highest occupied molecular orbital (HOMO, inset) of the NN-dative structure. ( b ) DOS of free pyridazine. The insets show pyridazine’s geometric structure and frontier orbitals. ( c ) Partial DOS curve of pyridazine of the N-dative structure, and the major frontier orbitals of the N-dative structure between −2 and 0 eV. The isovalue to plot the electron density isosurfaces of all orbitals is 1 × 10 −4 e Å −3 . The two vertical dash lines indicate the scanning tunnelling microscopy-resonating bias range from −2 to 0 eV. The energies refer to the valence band maximum of each model as zero. Full size image Figure 3c reveals that there are five small peaks of adsorbed pyridazine’s partial DOS of N-dative in the STM resonance range. The summed density of these five orbitals is less than one electron per unit cell, indicating that these peaks may originate from one frontier orbital of free pyridazine but are dispersed by surface states from the unreacted dimer atom. These orbitals are analogous in shape and also resemble the LUMO ( Fig. 3b ) of free pyridazine. However, four leaves of each orbital split into two groups, unlike the equivalent leaves in the LUMO of free pyridazine. The leaves from C 5 =C 6 (see C atom numbering in Fig. 2b ) are smaller than those from C 3 =C 4 . This difference is possibly due to the stronger interaction with the substrate because C 5 =C 6 is topologically closer to the binding N atom than C 3 =C 4 . These smaller leaves blurred into a large one under STM, presenting similar ‘clovers’ at biases −0.5 and −2.0 V. The dispersed orbitals indicate the LUMO orbital of pyridazine, although partially isolated from the surface, still electronically couples with the substrate states. The coupling should be attributed to the unreacted atom of the binding dimer because there is almost no interference from other dimers, as demonstrated in NN-dative. To completely decouple molecular orbitals from substrates, molecules with large binding/spacing groups could be designed to more effectively isolate the part to be imaged from the substrates [30] . Another strategy is to utilize bidentate rather than single bonds to completely eliminate both dangling bonds from the binding dimer, such as in NN-dative. We demonstrated for the first time that hybridized orbitals on clean semiconductor surfaces can be directly imaged by STM. Pyridazine molecules are adsorbed on Ge(100) through N–Ge single/double dative bond(s) in standing-up configurations. In these configurations, pyridazine partially isolates itself from the Ge(100) surface. The LUMO of free molecule is disturbed by surface states and becomes occupied on adsorption. However, the hybridized orbital is resolvable in filled-state STM images. The N–Ge dative bonds anchor pyridazine molecules to Ge(100) with good immobility and stability even at room temperature, which is viable for potential applications in molecule-based devices. We also demonstrated that the binding sites, binding mechanisms, orientations and electronic properties of molecules adsorbed on semiconductors could be reliably determined from orbital-resolved STM images. By carefully designing the molecules, this chemisorption strategy may be applied to many other reactive surfaces. Our work may inspire orbital resolving work in the study of chemisorbed molecules on clean semiconductors and other substrates. Equipments and sample preparation The experiments were performed in an ultra-high vacuum chamber with a base pressure of 1 × 10 −8 Pa. The chamber was equipped with an Omicron variable temperature STM and a high resolution electron energy loss spectrometer (LK-3000, LK Technologies). An OMICRON ultra-high vacuum chamber standard sample heater stage was mounted on a liquid nitrogen (N 2 ) cooled, Dewar-type sample holder, in the purposes of resistively annealing the sample and cooling it to 110 K. The sample used in the experiment was cut from an n -doped single-side polished Ge(100) wafer with a resistivity of 1–2 Ω cm and a size of 12 mm × 2 mm × 0.5 mm. The clean Ge surface was prepared by several cycles of 1,000 V Ar + sputtering and flashing to 1,000 K. Pyridazine (99%, Sigma-Aldrich) was purified via six freeze–pump–thaw cycles before being dosed onto the Ge(100) surface. STM and HREELS measurements STM tips were prepared by electrochemically etching tungsten wires. In STM experiments, the dosing was in situ during STM scanning, and the exposure was directly monitored by STM. For HREELS experiments, the electron beam with an energy of 6.0 eV impinged on the Ge(100) surface at an incident angle of 60° with a resolution of 60 cm −1 (full-width at half-maximum). The sample faced to the dosing tube aperture with a distance of 5 cm. The exposures were reported in the unit of Langmuir (1 Langmuir=10 −6 Torr s) without calibration of ion gauge sensitivity. DFT calculation The DFT calculations were performed using CASTEP in Materials Studio (version 5.5) of Accelrys [31] . Since the STM results show that the adsorption is not selective towards different reconstructions like 2 × 1, c(4 × 2) and p(2 × 2), thus a c(4 × 2) slab model of six layers was employed to simulate the clean Ge(100) surface, including four dimers on the surface, three layers in the middle and two frozen layers in their bulk positions at the bottom. The generalized gradient approximation with Perdew–Burke–Ernzerhof parameterizations [32] was employed to estimate the exchange-correlation effect. The kinetic energy cutoff was set at 330 eV. A 2 × 4 × 1 Monkhorst-Pack grid was used for Brillouin Zone sampling [33] . The force criteria for the converge of geometric optimization was 0.02 eV Å −1 . To simulate the STM images, we applied the Tersoff–Hamann approximation [8] . How to cite this article: He, J. H. et al. Orbital resolution of molecules covalently attached to a clean semiconductor surface. Nat. Commun. 5:3721 doi: 10.1038/ncomms4721 (2014).